Transcription factor IRF8 directs a silencing programme for TH17 cell differentiation T H 17 cells are recognized as a unique subset of T helper cells that have critical roles in the pathogenesis of autoimmunity and tissue inflammation. Although RORγt is necessary for the generation of T H 17 cells, the molecular mechanisms underlying the functional diversity of T H 17 cells are not fully understood. Here we show that a member of interferon regulatory factor (IRF) family of transcription factors, IRF8, has a critical role in silencing T H 17-cell differentiation. Mice with a conventional knockout, as well as a T cell-specific deletion, of the Irf8 gene exhibited more efficient T H 17 cells. Indeed, studies of an experimental model of colitis showed that IRF8 deficiency resulted in more severe inflammation with an enhanced T H 17 phenotype. IRF8 was induced steadily and inhibited T H 17-cell differentiation during T H 17 lineage commitment at least in part through its physical interaction with RORγt. These findings define IRF8 as a novel intrinsic transcriptional inhibitor of T H 17-cell differentiation. CD4 + T helper (T H ) T cell subsets are characterized by the secretion of unique cytokine profiles and have critical roles in orchestrating adaptive immune responses. In addition to T H 1 and T H 2 cells, T H 17 cells have been identified more recently as a third T H subset mediating inflammatory and autoimmune responses through the production of interleukin (IL)-17A, IL-17F and IL-22 (refs 1 , 2 , 3 , 4 ). T H 17 lineage commitment is initially driven by transforming growth factor (TGF)-β in the presence of IL-6 or IL-21 (refs 5 , 6 , 7 , 8 ), whereas IL-23 serves to expand or maintain T H 17 populations [2] , [5] , [9] , [10] . The orphan nuclear receptor, RORC, also known as RORγt, has been identified as the master transcription factor for T H 17 development [11] . The differentiation of T H 17 cells is also regulated by several recently described positive and negative feedback loops involving IL-21, IL-23R, IL-10 and IL-27 (refs 6 , 7 , 12 , 13 , 14 , 15 ), indicating that intrinsic genetic programmes may contribute to the silencing of T H 17 lineage commitment. There is, increasing evidence that T H 17 cells are involved in the pathogenesis of various autoimmune/inflammatory diseases, including multiple sclerosis, rheumatoid arthritis, inflammatory bowel diseases and asthma [16] . Thus, a more complete understating of the molecular mechanisms involved in the regulation of T H 17 immune responses should provide insights into the pathogenesis and treatment of these and possibly other inflammatory diseases. Several transcription factors, including RORγt, RORα, STAT3 and interferon regulatory factor (IRF)4, have been reported to be important for T H 17-cell differentiation. However, the silencing programme for T H 17-cell differentiation has not been fully examined. IRF8, a member of the IRF family, is expressed by B cells, dendritic cells (DCs), macrophages [17] , [18] , [19] and activated T cells [20] , [21] , and has been shown to have a diverse roles in the regulation of innate and adaptive immune responses. IRF8 has a DNA-binding domain in the amino (N)-terminal half of the protein and an IRF association domain in the carboxy (C) terminus that is responsible for heterodimerization with other transcription factors [22] . IRF8 functions as a transcriptional repressor or activator depending on the formation of different heterodimeric DNA-binding complexes with partners that include members of the ETS family and the IRF family [22] . It is known that IRF8 has critical roles in the differentiation of myeloid cells, promoting monocyte over granulocyte differentiation [23] . It is also a crucial regulator of many aspects of DC development, differentiation and function [24] , thereby having an essential role in the establishment of innate immune responses. Although IRF8 is critical for the regulation of immune cell growth, differentiation and survival [25] , the direct effects of IRF8 on T-cell activation and differentiation are incompletely understood. In the present study, we show that mice deficient in IRF8 because of a conventional knockout (KO) or with a T cell-specific conditional deletion exhibited enhanced T H 17-cell differentiation while exhibiting no significant effects on T H 1 or T H 2 cells. In addition, transfer of naive T cells from IRF8-deficient mice induced more severe colitis in Rag –/– mice than T cell from normal controls. Furthermore, we report that IRF8 physically interacts with RORγt, resulting in inhibition of IL-17 transcription. These findings suggest that IRF8 has a suppressive role in the control of T H 17 differentiation and highlight the importance of intrinsic genetic programmes for the silencing of T H 17-dependent immune responses. IRF8 deficiency enhances T H 17-cell differentiation To investigate the function of IRF8 in T cells, we first examined the expression of IRF8 in CD4 + T cells from normal or OT-II transgenic mice activated by different stimuli. We found that T-cell antigen receptor (TCR) engagement with anti-CD3 and anti-CD28 antibodies as well as stimulation of OT-II cells resulted in significant induction of IRF8 protein expression, as determined by western blotting ( Supplementary Fig. S1a,b ). Interestingly, IRF8 protein was more stably expressed in naive CD4 + T cells polarized for 12 to 72 h under T H 17-inducing conditions compared with T H 1- or T H 2-inducing conditions ( Supplementary Fig. S1a ). To clarify how T H 17-polarizing conditions induce stable IRF8 expression, CD4 + cells were stimulated with TGF-β in the absence of TCR activation and the results showed that TGF-β clearly induced IRF8 expression at both 48 and 72 h ( Supplementary Fig. S1c ). In addition, mitogen-activated protein kinase inhibitors significantly blocked IRF8 protein expression induced by TCR activation ( Supplementary Fig. S1d ) and STAT3 mutant mice showed impaired IRF8 mRNA expression ( Supplementary Fig. S1e ). These data indicate that IRF8 is consistently elevated in activated CD4 + T cells and TCR signalling cascade is involved in induction of IRF8 expression. We then assessed the contributions of IRF8 to T H 17 differentiation by studying CD4 + T cells from mice deficient in IRF8 due to a conventional KO of the gene ( Irf8 –/– mice). Naive CD4 + T cells from Irf8 –/– or wild-type (WT) littermate mice were primed in vitro for 4 days under T H 0 or T H 17 polarizing conditions. The cells were then re-stimulated with phorbol myristate acetate (PMA)/ionomycin and examined for the percentages of IL-17-producing cells by intracellular staining using flow cytometry. Notably, the frequency of IL-17-producing cells generated from Irf8 –/– T-cell cultures was about threefold greater than cells from WT cultures ( Fig. 1a ). These observations correlated with enhanced IL-17 secretion by Irf8 –/– T H cells generated under T H 17 polarizing conditions as determined by enzyme-linked immunosorbent assay (ELISA; Fig. 1b ). In addition, IL-17-producing CD4 + T cells were significantly increased among lamina propria lymphocytes isolated from Irf8 –/– mice as compared with WT littermate controls following in vitro activation under T H 17 conditions or at the basal levels ( Fig. 1c and Supplementary Fig. S2 ). 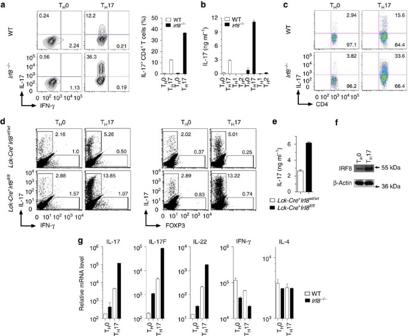Figure 1: Increased IL-17 production in IRF8 deficient T helper cells. (a) Naive CD4+T cells from wild-type (WT) orIrf8–/–mice were differentiated under TH0 and TH17 polarizing conditions for 4 days. Cells were then re-stimulated with PMA/ionomycin for 5 h, stained for intracellular IL-17 and IFN-γ, and analysed by flow cytometry. Representative fluorescence-activated cell sorting (FACS) dot plots gated on CD4+cells and the percentages of IL-17-producing CD4+cells are shown. Data are from one experiment representative of three independent experiments. Error bars, s.d. (b) The cells prepared ina, TH1 and TH2 polarizing conditions were re-stimulated with PMA/ionomycin for 24 h and the supernatants were analysed for IL-17 by ELISA. Data are from one experiment representative of three independent experiments. Error bars, s.d. (c) Wild-type orIrf8–/–lamina propria lymphocytes (LPL) were differentiated under TH17 conditions for 4 days. Cells were then re-stimulated with PMA/ionomycin for 5 h, stained for intracellular IL-17 and analysed by flow cytometry. (d) Naive CD4+T cells fromLck-Cre+Irf8wt/wtandLck-Cre+Irf8fl/flmice were differentiated under TH0 and TH17 polarizing conditions for 4 days and the cells were re-stimulated with PMA/ionomycin for 5 h for staining of IL-17, IFN-γ and FOXP3. Representative FACS dot plots gated on CD4+cells are shown. (e) The cells prepared indwere re-stimulated with PMA/ionomycin for 24 h and the supernatants were analysed for IL-17 by ELISA. Data are from one experiment representative of two independent experiments. Error bars, s.d. (f) Naive CD4+T cells from C57BL/6 mice were differentiated under TH0 and TH17 conditions for 4 days. The cells were re-stimulated with PMA/ionomycin for 12 h and IRF8 expression was analysed by western blot. (g) The cells prepared inawere re-stimulated with PMA/ionomycin for 5 h and mRNA expression of indicated genes was determined by qPCR. The data shown were normalized to levels of ubiquitin expression as analysed by qPCR. The results are representative of three independent experiments. Error bars, s.d. Figure 1: Increased IL-17 production in IRF8 deficient T helper cells. ( a ) Naive CD4 + T cells from wild-type (WT) or Irf8 –/– mice were differentiated under T H 0 and T H 17 polarizing conditions for 4 days. Cells were then re-stimulated with PMA/ionomycin for 5 h, stained for intracellular IL-17 and IFN-γ, and analysed by flow cytometry. Representative fluorescence-activated cell sorting (FACS) dot plots gated on CD4 + cells and the percentages of IL-17-producing CD4 + cells are shown. Data are from one experiment representative of three independent experiments. Error bars, s.d. ( b ) The cells prepared in a , T H 1 and T H 2 polarizing conditions were re-stimulated with PMA/ionomycin for 24 h and the supernatants were analysed for IL-17 by ELISA. Data are from one experiment representative of three independent experiments. Error bars, s.d. ( c ) Wild-type or Irf8 –/– lamina propria lymphocytes (LPL) were differentiated under T H 17 conditions for 4 days. Cells were then re-stimulated with PMA/ionomycin for 5 h, stained for intracellular IL-17 and analysed by flow cytometry. ( d ) Naive CD4 + T cells from Lck-Cre + Irf8 wt/wt and Lck-Cre + Irf8 fl/fl mice were differentiated under T H 0 and T H 17 polarizing conditions for 4 days and the cells were re-stimulated with PMA/ionomycin for 5 h for staining of IL-17, IFN-γ and FOXP3. Representative FACS dot plots gated on CD4 + cells are shown. ( e ) The cells prepared in d were re-stimulated with PMA/ionomycin for 24 h and the supernatants were analysed for IL-17 by ELISA. Data are from one experiment representative of two independent experiments. Error bars, s.d. ( f ) Naive CD4 + T cells from C57BL/6 mice were differentiated under T H 0 and T H 17 conditions for 4 days. The cells were re-stimulated with PMA/ionomycin for 12 h and IRF8 expression was analysed by western blot. ( g ) The cells prepared in a were re-stimulated with PMA/ionomycin for 5 h and mRNA expression of indicated genes was determined by qPCR. The data shown were normalized to levels of ubiquitin expression as analysed by qPCR. The results are representative of three independent experiments. Error bars, s.d. Full size image To determine whether the effects of IRF8 deficiency on T H 17 potential were cell type-specific, we next compared CD4 + T cells from mice expressing Lck-Cre that were WT (wt/wt) or homozygous ( fl/fl ) for a conditional allele of Irf8 gene resulting in selective depletion of IRF8 in the T-cell compartment. Quantitative real-time reverse transcrption(RT)–PCR (qPCR) analyses revealed dramatically lower levels of Irf8 transcripts in sorted thymocyte sub-populations (DP, CD4SP, CD8SP) and splenic CD3 + CD4 + cells from Lck-Cre + Irf8 fl/fl compared with cells from Lck-Cre + Irf8 wt/wt littermate control mice ( Supplementary Fig. S3 ), confirming that the Irf8 gene was efficiently deleted from Lck-Cre + Irf8 fl/fl T cells. Splenic and lymph node CD4 + T-cell subsets from mice with IRF8-deficient T cells as well as from mice homozygous for a conventional Irf8 null allele were normal in number as well as in expression of the T-cell activation markers CD62L, CD44, CD25 and CD69. Expression of FOXP3 in thymic and peripheral lymph node T cells from mice of both genotypes was also similar ( Supplementary Fig. S4 ), indicating that CD4 + T cells develop normally in the absence of IRF8. Naive CD4 + T cells from Lck-Cre + Irf8 fl/fl and Lck-Cre + Irf8 wt/wt littermate controls were subjected to T H 17 polarization. As expected, T H cells from mice with a T cell-specific deficiency in IRF8 showed a remarkable increase in the generation of IL-17-producing cells ( Fig. 1d ) in association with significantly elevated levels of IL-17 secretion ( Fig. 1e ). These results excluded the possibility that the effects of IRF8 deficiency on T cells from mice with a conventional KO of the gene could be attributed to the altered activities of other subsets of IRF8-deficient cells, such as B cells, DC or macrophages. T H 17 cells generated from splenic T cells of Irf8 –/– mice comprised a major portion of the β-TCR + CD4 + lymphocyte subset ( Supplementary Fig. S5 ). Indeed, high levels of IRF8 protein expression were detected in CD4 + T cells polarized under T H 17 conditions as determined by immunoblot analyses ( Fig. 1f ). Accordingly, transcript levels of the iconic T H 17 cytokines IL-17A, IL-17F and IL-22 were enhanced in Irf8 –/– T H 17 cells ( Fig. 1g ). In contrast, T H 1 or T H 2 differentiation was not noticeably affected in Irf8 –/– T-cell cultures ( Fig. 2a–c ). In addition, [ 3 H]-Thymidine incorporation assay showed that the proliferation of CD4 + T cells from Lck-Cre + Irf8 fl/fl and Lck-Cre + Irf8 wt/wt mice cultured under T H 17 conditions was comparable ( Fig. 2d ). Taken together, these results indicate that IRF8 is induced during T-cell activation, and that T H 17-cell differentiation is enhanced in cells deficient in IRF8. 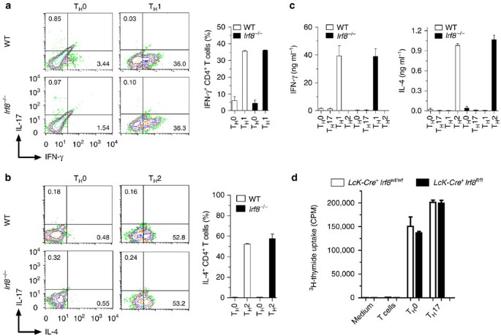Figure 2: TH1 and TH2 differentiation inIrf8–/–CD4+T cells. Naive CD4+T cells of WT orIrf8–/–mice were differentiated under TH1 or TH2 polarizing conditions for 4 days. Cells were then re-stimulated with PMA/ionomycin for 5 h and stained for intracellular IFN-γ as a TH1 marker (a) and IL-4 as a TH2 marker (b) by flow cytometry. Data are from one experiment representative of three independent experiments. Error bars, s.d. The cells prepared inaandbwere re-stimulated with PMA/ionomycin for 12 h and the supernatants were analysed for IFN-γ and IL-4 by ELISA (c). Data are from one experiment representative of three independent experiments. Error bars, s.d. Naive CD4+T cells from spleens and lymph nodes ofLck-Cre+Irf8wt/wtandLck-Cre+Irf8fl/flmice were prepared and the cells were differentiated under TH0 and TH17 polarizing conditions for 3 days. [3H]-Thymidine was added during the last 8 h of culture. Then the cells were collected and were counted with a beta-counter (d). Data are from one experiment representative of two independent experiments. Error bars, s.d. Figure 2: T H 1 and T H 2 differentiation in Irf8 –/– CD4 + T cells. Naive CD4 + T cells of WT or Irf8 –/– mice were differentiated under T H 1 or T H 2 polarizing conditions for 4 days. Cells were then re-stimulated with PMA/ionomycin for 5 h and stained for intracellular IFN-γ as a T H 1 marker ( a ) and IL-4 as a T H 2 marker ( b ) by flow cytometry. Data are from one experiment representative of three independent experiments. Error bars, s.d. The cells prepared in a and b were re-stimulated with PMA/ionomycin for 12 h and the supernatants were analysed for IFN-γ and IL-4 by ELISA ( c ). Data are from one experiment representative of three independent experiments. Error bars, s.d. Naive CD4 + T cells from spleens and lymph nodes of Lck-Cre + Irf8 wt/wt and Lck-Cre + Irf8 fl/fl mice were prepared and the cells were differentiated under T H 0 and T H 17 polarizing conditions for 3 days. [ 3 H]-Thymidine was added during the last 8 h of culture. Then the cells were collected and were counted with a beta-counter ( d ). Data are from one experiment representative of two independent experiments. Error bars, s.d. Full size image T reg cells and autocrine cytokines are not altered in Irf8 –/– mice To understand whether alterations in T reg cells might contribute to enhanced T H 17 differentiation in IRF8-deficient mice, we analysed FOXP3 + CD4 + T cells in these mice. There were no significant differences between the FOXP3 + CD4 + T-cell populations of WT and Irf8 –/– mice under T H 17- or T reg -inducing conditions ( Fig. 3a,b ). Thus, the more efficient generation of Irf8 –/– T H 17 cells in response to the combined effects of TGF-β plus IL-6 was not because of alterations in TGF-β-derived T reg suppression. IL-17-producing cells generated from Irf8 –/– T-cell cultures were greatly increased following stimulation with IL-6 plus TGF-β ( Fig. 3c ). 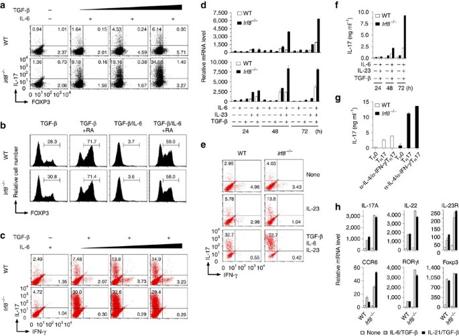Figure 3: IRF8 inhibits the expression of TH17-associated genes. Naive CD4+T cells from wild-type andIrf8–/–mice were stimulated with plate-bound anti-CD3 and anti-CD28 antibodies in the presence of IL-6 (10 ng ml−1) plus differing concentrations of TGF-β (0.1, 1, 5 ng ml−1) (a), or TGF-β (5 ng ml−1), TGF-β (5 ng ml−1)/IL-6 (10 ng ml−1) with or without retinoic acid (RA, 100 nM) (b). After 4 days of stimulation, IL-17 and FOXP3 intracellular staining was performed and analysed by flow cytometry. (c) The cells prepared inaandbexcept for the presence of TGF-β (5 ng ml−1) plus various concentrations of IL-6 (5, 10, 50, 100 ng ml−1) were re-stimulated with PMA/ionomycin for 5 h and stained for intracellular IL-17 and IFN-γ and analysed by flow cytometry. (d) Naive CD4+T cells from wild-type andIrf8–/–mice were stimulated with IL-6, IL-23, TGF-β or different combinations of these cytokines for various intervals. Total RNA was extracted and analysed by RT–PCR for mRNA expression of IL-17 (top panel) and IL-17F (bottom panel). Data are from one experiment representative of three independent experiments. Error bars, s.d. (e) Naive CD4+T cells from WT andIrf8–/–mice were stimulated with the indicated cytokines for 4 days. Cells were re-stimulated with PMA/ionomycin for 5 h and stained for intracellular IL-17 and IFN-γ and analysed by flow cytometry. The results are representative of three independent experiments. (f) Cells were prepared as ineand the culture supernatants were collected after 4 days of stimulation. IL-17 protein secretion was analysed by ELISA. (g) Naive CD4+T cells from WT andIrf8–/–mice were prepared and stimulated with TGF-β and IL-6 in the presence of neutralizing anti-IFN-γ (10 μg ml−1) and anti-IL-4 (10 μg ml−1) antibodies. At 72 h after the stimulation, IL-17 protein secretion in culture supernatants was analysed by ELISA. Data are the mean±s.d. of triplicate cultures. (h) Naive CD4+T cells from wild-type orIrf8–/–mice were stimulated with the indicated cytokine combinations for 48 h. Total RNA was extracted and analysed by qPCR for mRNA expression of the indicated genes. Data are from one experiment representative of three independent experiments. Error bars, s.d. Figure 3: IRF8 inhibits the expression of T H 17-associated genes. Naive CD4 + T cells from wild-type and Irf8 –/– mice were stimulated with plate-bound anti-CD3 and anti-CD28 antibodies in the presence of IL-6 (10 ng ml −1 ) plus differing concentrations of TGF-β (0.1, 1, 5 ng ml −1 ) ( a ), or TGF-β (5 ng ml −1 ), TGF-β (5 ng ml −1 )/IL-6 (10 ng ml −1 ) with or without retinoic acid (RA, 100 nM) ( b ). After 4 days of stimulation, IL-17 and FOXP3 intracellular staining was performed and analysed by flow cytometry. ( c ) The cells prepared in a and b except for the presence of TGF-β (5 ng ml −1 ) plus various concentrations of IL-6 (5, 10, 50, 100 ng ml −1 ) were re-stimulated with PMA/ionomycin for 5 h and stained for intracellular IL-17 and IFN-γ and analysed by flow cytometry. ( d ) Naive CD4 + T cells from wild-type and Irf8 –/– mice were stimulated with IL-6, IL-23, TGF-β or different combinations of these cytokines for various intervals. Total RNA was extracted and analysed by RT–PCR for mRNA expression of IL-17 (top panel) and IL-17F (bottom panel). Data are from one experiment representative of three independent experiments. Error bars, s.d. ( e ) Naive CD4 + T cells from WT and Irf8 –/– mice were stimulated with the indicated cytokines for 4 days. Cells were re-stimulated with PMA/ionomycin for 5 h and stained for intracellular IL-17 and IFN-γ and analysed by flow cytometry. The results are representative of three independent experiments. ( f ) Cells were prepared as in e and the culture supernatants were collected after 4 days of stimulation. IL-17 protein secretion was analysed by ELISA. ( g ) Naive CD4 + T cells from WT and Irf8 –/– mice were prepared and stimulated with TGF-β and IL-6 in the presence of neutralizing anti-IFN-γ (10 μg ml −1 ) and anti-IL-4 (10 μg ml −1 ) antibodies. At 72 h after the stimulation, IL-17 protein secretion in culture supernatants was analysed by ELISA. Data are the mean±s.d. of triplicate cultures. ( h ) Naive CD4 + T cells from wild-type or Irf8 –/– mice were stimulated with the indicated cytokine combinations for 48 h. Total RNA was extracted and analysed by qPCR for mRNA expression of the indicated genes. Data are from one experiment representative of three independent experiments. Error bars, s.d. Full size image To further investigate how IRF8 affects T H 17 differentiation, naive WT and Irf8 –/– CD4 + T cells were subjected to T H 17 differentiation in the presence of IL-6, IL-23 and TGF-β, either alone or in various combinations, and then examined for the expression of lineage-specific genes by qPCR. Neither IL-6 nor TGF-β alone induced significant levels of IL-17 or IL-17F transcripts ( Fig. 3d ). In contrast, dramatic increases in IL-17 and IL-17F transcripts were induced at multiple time points by the combination of IL-23, IL-6 and TGF-β in cultures of both Irf8 –/– and WT T cells ( Fig. 3d ). Increased expression of IL-17 was confirmed at the protein level by ELISA ( Fig. 3e–g ). IL-23 induced low levels of IL-17 and IL-17F transcripts with no significant differences being seen between CD4 + T cells of WT and Irf8 –/– mice ( Fig. 3d ). This suggests that IRF8 may not target the IL-23 signalling cascade, but may exert a major influence on T H 17 differentiation instead of T H 17 expansion and maintenance. IL-21, an autocrine cytokine produced by CD4 + T follicular helper cells and T H 17 cells [6] , [7] , induces T H 17 differentiation in the presence of TGF-β. IRF8-deficient T cells displayed enhanced induction of T H 17-associated molecules following stimulation by TGF-β combined with IL-6 or IL-21 ( Figs 3h and 4a ). However, production of IL-21 and IL-10 was comparable in WT and Irf8 –/– T H 17 cells ( Fig. 4b–e ). These results suggest that an autocrine loop involving either IL-21 or IL-10 is not involved in the functional control of T H 17 differentiation by IRF8. 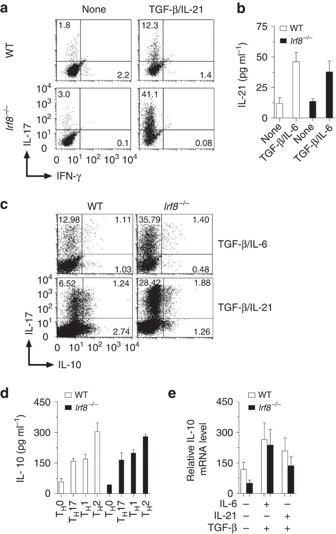Figure 4: IL-21 signalling and IL-10 production during TH17-cell differentiation inIrf8–/–mice. Naive CD4+T cells from WT andIrf8–/–mice were prepared, and the cells were stimulated with anti-CD3 and anti-CD28 antibodies in the presence or absence of TGF-β plus IL-21 or IL-6 for 72 h. Intracellular staining for IL-17 and IFN-γ expression was performed and analysed by flow cytometry (a). The secretion of IL-21 protein in culture supernatants was analysed by ELISA (b). Data are from one experiment representative of three independent experiments. Error bars, s.d. Naive CD4+T cells were stimulated with anti-CD3 and anti-CD28 antibodies in the presence of TGF-β plus IL-6 or IL-21. At 96 h after stimulation, intracellular staining for IL-17 and IL-10 was performed and analysed after re-stimulation with PMA/ionomycin by flow cytometry (c). Naive CD4+T cells from spleens and lymph nodes of WT andIrf8–/–mice were prepared and the cells were stimulated under TH0, TH1, TH2 and TH17 polarizing conditions for 4 days. Then the cells were re-stimulated with PMA/ionomycin for 12 h and IL-10 protein secretion was analysed by ELISA (d). Data are from one experiment representative of three independent experiments. Error bars, s.d. Naive CD4+T cells were stimulated with anti-CD3 and anti-CD28 antibodies in the presence of TGF-β plus IL-6 or IL-21 for 72 h. IL-10 expression was analysed by RT–PCR (e). Data are from one experiment representative of three independent experiments. Error bars, s.d. Figure 4: IL-21 signalling and IL-10 production during T H 17-cell differentiation in Irf8 –/– mice. Naive CD4 + T cells from WT and Irf8 –/– mice were prepared, and the cells were stimulated with anti-CD3 and anti-CD28 antibodies in the presence or absence of TGF-β plus IL-21 or IL-6 for 72 h. Intracellular staining for IL-17 and IFN-γ expression was performed and analysed by flow cytometry ( a ). The secretion of IL-21 protein in culture supernatants was analysed by ELISA ( b ). Data are from one experiment representative of three independent experiments. Error bars, s.d. Naive CD4 + T cells were stimulated with anti-CD3 and anti-CD28 antibodies in the presence of TGF-β plus IL-6 or IL-21. At 96 h after stimulation, intracellular staining for IL-17 and IL-10 was performed and analysed after re-stimulation with PMA/ionomycin by flow cytometry ( c ). Naive CD4 + T cells from spleens and lymph nodes of WT and Irf8 –/– mice were prepared and the cells were stimulated under T H 0, T H 1, T H 2 and T H 17 polarizing conditions for 4 days. Then the cells were re-stimulated with PMA/ionomycin for 12 h and IL-10 protein secretion was analysed by ELISA ( d ). Data are from one experiment representative of three independent experiments. Error bars, s.d. Naive CD4 + T cells were stimulated with anti-CD3 and anti-CD28 antibodies in the presence of TGF-β plus IL-6 or IL-21 for 72 h. IL-10 expression was analysed by RT–PCR ( e ). Data are from one experiment representative of three independent experiments. Error bars, s.d. Full size image We next determined whether the induction of T H 17-associated genes may be affected by forced expression of IRF8 in T cells. Retroviral transduction of IRF8-IRES-GFP into WT naive CD4 + T cells significantly decreased the percentage of IL-17-producing cells under T H 17 polarizing conditions ( Fig. 5a ), and RORγt-positive cells were moderately reduced ( Fig. 5a ). Similarly, retroviral transduction of IRF8 into the EL4T lymphoma cell line stimulated with PMA/ionomycin resulted in significantly reduced transcripts for IL-17, but had no effect on the expression of interferon (IFN)-γ, IL-4, IL-10 or FOXP3 ( Fig. 5b ). Taken together, these results demonstrate a direct role for IRF8 in suppressing T H 17-specific gene expression. 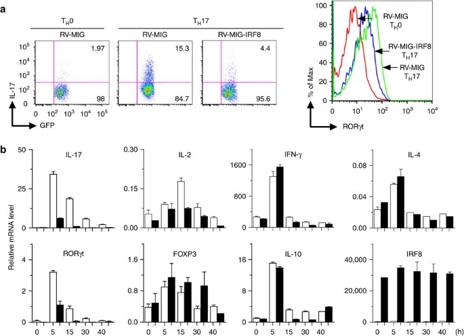Figure 5: Transduction of IRF8 inhibits TH17-associated genes. (a) Naive CD4+T cells from C57BL/6 mice were infected with retrovirus encoding IRF8 or empty vector and were activated under TH17-inducing conditions for 4 days. The cells were re-stimulated with PMA/ionomycin for 5 h and stained for intracellular IL-17 and RORγt and analysed by flow cytometry. (b) EL4 cells were transduced with retroviruses encoding IRF8 (black column) or GFP (white column) for 48 h and the transduced cells were then stimulated with PMA/ionomycin for various times as indicated. Total RNA was extracted and the transcript levels of TH17-associated genes were analysed by qPCR as indicated. The results are normalized to ubiquitin levels. Data are from one experiment representative of three independent experiments. Error bars, s.d. Figure 5: Transduction of IRF8 inhibits T H 17-associated genes. ( a ) Naive CD4 + T cells from C57BL/6 mice were infected with retrovirus encoding IRF8 or empty vector and were activated under T H 17-inducing conditions for 4 days. The cells were re-stimulated with PMA/ionomycin for 5 h and stained for intracellular IL-17 and RORγt and analysed by flow cytometry. ( b ) EL4 cells were transduced with retroviruses encoding IRF8 (black column) or GFP (white column) for 48 h and the transduced cells were then stimulated with PMA/ionomycin for various times as indicated. Total RNA was extracted and the transcript levels of T H 17-associated genes were analysed by qPCR as indicated. The results are normalized to ubiquitin levels. Data are from one experiment representative of three independent experiments. Error bars, s.d. Full size image IRF8 interacts with RORγt and suppresses IL-17 transcription The above findings prompted us to probe the molecular basis for IRF8 control of T H 17-cell differentiation. As many studies have demonstrated a critical role for RORγt in T H 17-cell differentiation both in vitro and in vivo [11] , we asked if IRF8 might affect RORγt-mediated IL-17 induction. EL4 cells were transiently transfected RORγt followed by stimulation with PMA/ionomycin. Overexpression of RORγt resulted in significantly increased expression of IL-17 and IL-17F, whereas co-transfection with IRF8 greatly reduced the expression of these genes, suggesting that IRF8 inhibits RORγt-induced expression of IL-17 transcripts ( Fig. 6a ). Using a 6-kbp IL-17 promoter reporter plasmid, we confirmed that RORγt strongly induced IL-17 promoter reporter activity in 293T cells ( Fig. 6b ), which was shown to be due to a direct effect of RORγt on the IL-17 promoter [26] , [27] . Co-transfection of IRF8 in these cells suppressed RORγt-mediated IL-17 promoter activity in a dose-dependent manner ( Fig. 6c ). Similar results were observed in EL4 cells ( Fig. 6d ). CNS2 is a conserved non-coding sequence (CNS) element ∼ 5 kbp upstream of the IL-17 locus that functions as a RORγt-dependent enhancer element required for optimal IL-17 transcription [27] , [28] . Overexpression of IRF8 significantly suppressed CNS2-enhanced IL-17 promoter activity ( Fig. 6e ), indicating that IRF8 inhibits IL-17 transcription. 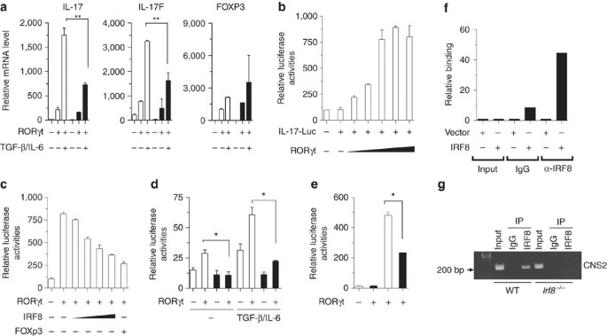Figure 6: IRF-8 represses IL-17 transcription. (a) IRF8-expressing EL4 cells (black column) or control cells (white column) were transiently transfected with a RORγt plasmid for 24 h, and the cells were treated with plate-bound anti-CD3 and anti-CD28 antibodies in the presence or absence of the indicated cytokines for 8 h. qPCR analyses of transcripts of the indicated genes were performed and the results were normalized to the levels of ubiquitin transcripts. **P<0.01 versus cells transfected with IRF8 (Student'st-test). Data are representative of multiple experiments. (b) 293T cells were co-transfected with an IL-17 promoter reporter construct containing a 6-kbp promoter and increasing doses of a RORγt plasmid for 30 h. (c) 293T cells were co-transfected with an IL-17 promoter reporter construct containing a 6-kbp promoter, a RORγt plasmid, a FOXP3 plasmid, and increasing doses of an IRF8 plasmid for 30 h. (d) IRF8-expressing EL4 cells (black column) or control cells (white column) were co-transfected with an IL-17 promoter reporter construct containing a 6-kbp promoter plus RORγt plasmid, and treated with plate-bound anti-CD3 antibody in the presence or absence of the indicated cytokines for 24 h. Luciferase activities in (b,c,d) were measured and normalized to β-galactosidase activity. Data are mean±s.d. of triplicate cultures and are representative of three independent experiments. *P<0.05 versus cells transfected with IRF8 (Student'st-test). (e) IRF8-expressing EL4 cells (black column) or control cells (white column) were co-transfected with an IL-17 promoter reporter construct containing a minimal 1.1-kb promoter plus CNS2, and RORγt plasmids. The cells were treated with plate-bound anti-CD3 and anti-CD28 antibodies and IL-6/TGF-β for 24 h. A luciferase assay was performed as described in (b), (c), and (d). *P<0.05 versus cells transfected with IRF8 (Student'st-test). (f) 293T cells were co-transfected with an IL-17 promoter reporter construct (containing CNS2) with either an IRF8 overexpression plasmid or a control vector for 36 h, followed by ChIP analysis. 3 μg of anti-IRF8 antibody or isotype-matched IgG as control antibody were used in the immunoprecipitation step. qPCR was used to quantify the amount of precipitated DNA with primers flanking the CNS2 region of the IL-17 promoter. Data were normalized to input DNA in each respective sample. (g) Naive CD4+T cells from wild-type orIrf8–/–mice were cultured under TH17-polarizing conditions for 60 h, followed by ChIP assay as described above. 3 μg of anti-IRF8 antibody or isotype-matched IgG as control antibody were used in the immunoprecipitation step. PCR was used to quantify the amount of precipitated DNA with primers flanking the CNS2 region of the IL-17 promoter. Figure 6: IRF-8 represses IL-17 transcription. ( a ) IRF8-expressing EL4 cells (black column) or control cells (white column) were transiently transfected with a RORγt plasmid for 24 h, and the cells were treated with plate-bound anti-CD3 and anti-CD28 antibodies in the presence or absence of the indicated cytokines for 8 h. qPCR analyses of transcripts of the indicated genes were performed and the results were normalized to the levels of ubiquitin transcripts. ** P <0.01 versus cells transfected with IRF8 (Student's t -test). Data are representative of multiple experiments. ( b ) 293T cells were co-transfected with an IL-17 promoter reporter construct containing a 6-kbp promoter and increasing doses of a RORγt plasmid for 30 h. ( c ) 293T cells were co-transfected with an IL-17 promoter reporter construct containing a 6-kbp promoter, a RORγt plasmid, a FOXP3 plasmid, and increasing doses of an IRF8 plasmid for 30 h. ( d ) IRF8-expressing EL4 cells (black column) or control cells (white column) were co-transfected with an IL-17 promoter reporter construct containing a 6-kbp promoter plus RORγt plasmid, and treated with plate-bound anti-CD3 antibody in the presence or absence of the indicated cytokines for 24 h. Luciferase activities in ( b , c , d ) were measured and normalized to β-galactosidase activity. Data are mean±s.d. of triplicate cultures and are representative of three independent experiments. * P <0.05 versus cells transfected with IRF8 (Student's t -test). ( e ) IRF8-expressing EL4 cells (black column) or control cells (white column) were co-transfected with an IL-17 promoter reporter construct containing a minimal 1.1-kb promoter plus CNS2, and RORγt plasmids. The cells were treated with plate-bound anti-CD3 and anti-CD28 antibodies and IL-6/TGF-β for 24 h. A luciferase assay was performed as described in ( b ), ( c ), and ( d ). * P <0.05 versus cells transfected with IRF8 (Student's t -test). ( f ) 293T cells were co-transfected with an IL-17 promoter reporter construct (containing CNS2) with either an IRF8 overexpression plasmid or a control vector for 36 h, followed by ChIP analysis. 3 μg of anti-IRF8 antibody or isotype-matched IgG as control antibody were used in the immunoprecipitation step. qPCR was used to quantify the amount of precipitated DNA with primers flanking the CNS2 region of the IL-17 promoter. Data were normalized to input DNA in each respective sample. ( g ) Naive CD4 + T cells from wild-type or Irf8 –/– mice were cultured under T H 17-polarizing conditions for 60 h, followed by ChIP assay as described above. 3 μg of anti-IRF8 antibody or isotype-matched IgG as control antibody were used in the immunoprecipitation step. PCR was used to quantify the amount of precipitated DNA with primers flanking the CNS2 region of the IL-17 promoter. Full size image To investigate whether IRF8 can directly bind the CNS2 region of the IL-17 promoter, we co-transfected an IL-17 promoter reporter (containing CNS2) and IRF8 plasmids into 293T cells and performed chromatin immunoprecipitation (ChIP) using an IRF8-specific antibody. The precipitated chromatin DNA was analysed by qPCR using primers covering the CNS2 region of the IL-17 promoter. The results showed that IRF8 antibody specifically pulled down the CNS2 region sequences ( Fig. 6f ). To confirm the results, naive WT and Irf8 –/– CD4 + T cells were stimulated under T H 17 polarizing conditions for 60 h and ChIP assay was performed as above. The precipitated chromatin DNA was analysed by PCR using primers covering the CNS2 region of the IL-17 promoter. Similarly, IRF8 antibody specifically pulled down the CNS2 region sequences of T H 17 cells from WT mice but not from Irf8 –/– mice ( Fig. 6g ). These results demonstrate that IRF8 bound directly to this region of the IL-17 promoter. Further analyses of the CNS2 sequence revealed several IRF consensus binding sequence elements ( Supplementary Fig. S6a ). We showed that mutation of a typical IRF-binding site in the CNS2 region of IL-17 promoter nullified the inhibition of RORγt-mediated IL-17 promoter activation by IRF8 ( Supplementary Fig. S6b ). These results provided a molecular basis for understanding the inhibitory effects of IRF8 on IL-17 transcription. It is likely that RORγt cooperates with other known transcription factors, such as FOXP3 or RUNX1, or unknown factors in the coordinate regulation of T H 17 differentiation [26] , [29] , [30] . We then co-transfected HA-tagged IRF8 and T7-RORγt plasmids into 293T cells for co-immunoprecipitation. Immunoprecipitation of RORγt resulted in co-precipitation of IRF8 ( Fig. 7a ), even in the presence of ethidium bromide or DNase I, indicating that IRF8 and RORγt interact with each other without the involvement of DNA. Using confocal microscopy, we also determined that IRF8 and RORγt co-localized in the nucleus of NIH3T3 cells co-transfected with GFP-IRF8 and T7-RORγt constructs ( Fig. 7b ). Flow cytometric analyses of naive CD4 + T cells stimulated under T H 17 polarizing conditions clearly revealed a population of RORγt + CD4 + cells with the majority of these cells also staining for IRF8 ( Fig. 7c ). Furthermore, anti-IRF8 antibodies were found to co-immunoprecipitate RORγt from lysates of primary CD4 + T cells from WT but not from Irf8 –/– mice cultured under T H 17 polarizing conditions ( Fig. 7d ), indicating that endogenous IRF8 and RORγt interact with each other. 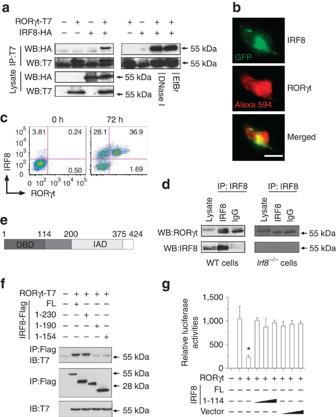Figure 7: IRF8 interacts physically with RORγ. (a) 293T cells were transfected with HA-tagged IRF8 and T7-tagged RORγt overexpression plasmids for 40 h and cell lysates were prepared in the presence or absence of DNase I or ethidium bromide. 500 μg of cell lysates were immunoprecipitated with an anti-T7 antibody and immunoblotted with specific antibodies as indicated. Data are representative of three independent experiments. (b) NIH3T3 cells were transiently transfected with GFP-IRF8 and T7-RORγt for 40 h, and cells were fixed and stained red for RORγt followed by confocal microscopic analysis. Scale bar, 50 μm. (c) Naive CD4+T cells from WT mice were cultured under TH17-polarizing conditions for 72 h and the expression of RORγt and IRF8 was analysed by flow cytometry. The cells were gated on CD4+T cells. Data are representative of three independent experiments. (d) Naive CD4+T cells from wild-type orIrf8–/–mice were cultured under TH17-polarizing conditions for 60 h and the cell lysates were then immunoprecipitated with an anti-IRF8 antibody and western blotted (WB) with anti-RORγt and anti-IRF8 antibodies. Data represent three independent experiments. (e) Diagrams of IRF8 protein domains. (f) 293T cells were co-transfected with plasmids containing Flag-tagged full-length IRF8, IRF8 fragments (1–230, 1–190, 1–154) and T7-tagged RORγt plasmid for 40 h, and co-immunoprecipitation using anti-Flag antibody from the cell extracts was performed and immunoblotted with anti-T7 antibody. Data are representative of three independent experiments. (g) 293T cells were co-transfected with an IL-17 promoter reporter construct containing the 6-kbp promoter, a RORγt plasmid and either a full-length IRF8 or the IRF8 truncation mutant (1–114) construct for 30 h. Luciferase assays were performed as described inb. Data indicate mean±s.d. of triplicate cultures and are representative of three independent experiments. *P<0.05 versus cells transfected with IRF8 mutant (Student'st-test). As shown in Figure 7e , IRF8 is comprised of an N-terminal DNA-binding domain, a flanking internal region, and a C-terminal IRF association domain [31] . To map the binding sites between IRF8 on RORγt, we co-transfected 293T cells with T7-tagged RORγt and Flag-tagged full-length IRF8 or one of a series of C-terminal truncation mutants (1–390, 1–356, 1–305, 1–253, 1–230, 1–190 and 1–154) followed by co-immunoprecipitation experiments. The results showed that IRF8 amino-acid residues between 230 and 190 were important for the physical interaction with RORγt ( Supplementary Fig. S7a , Fig. 7f ). IRF8 mutant (1–114), which is not bound to RORγt, did not suppress RORγt-mediated IL-17 promoter activation as WT and other binding mutants did ( Fig. 7g and Supplementary Fig. S7b ), demonstrating that the inhibitory activity of IRF8 on IL-17 transcription is related to its interaction with RORγt. In addition, IRF4, another IRF family member that is required for the generation of T H 17 cells [32] , was also found in co-immunoprecipitation experiments to interact with RORγt, whereas there was no interaction between IRF1 and RORγt ( Supplementary Fig. S8a ). Although transcript levels for IRF4 in cells deficient in IRF8 did not change under T H 17 polarizing conditions ( Supplementary Fig. S8b ), we still cannot exclude possibility that IRF8 and IRF4 mutually influence their activities in T H 17 cells. Thus, our results suggest that protein–protein interactions between IRF8 and RORγt have at least a partial role in IRF8-mediated inhibitory effects on IL-17 transcription. Figure 7: IRF8 interacts physically with RORγ. ( a ) 293T cells were transfected with HA-tagged IRF8 and T7-tagged RORγt overexpression plasmids for 40 h and cell lysates were prepared in the presence or absence of DNase I or ethidium bromide. 500 μg of cell lysates were immunoprecipitated with an anti-T7 antibody and immunoblotted with specific antibodies as indicated. Data are representative of three independent experiments. ( b ) NIH3T3 cells were transiently transfected with GFP-IRF8 and T7-RORγt for 40 h, and cells were fixed and stained red for RORγt followed by confocal microscopic analysis. Scale bar, 50 μm. ( c ) Naive CD4 + T cells from WT mice were cultured under T H 17-polarizing conditions for 72 h and the expression of RORγt and IRF8 was analysed by flow cytometry. The cells were gated on CD4 + T cells. Data are representative of three independent experiments. ( d ) Naive CD4 + T cells from wild-type or Irf8 –/– mice were cultured under T H 17-polarizing conditions for 60 h and the cell lysates were then immunoprecipitated with an anti-IRF8 antibody and western blotted (WB) with anti-RORγt and anti-IRF8 antibodies. Data represent three independent experiments. ( e ) Diagrams of IRF8 protein domains. ( f ) 293T cells were co-transfected with plasmids containing Flag-tagged full-length IRF8, IRF8 fragments (1–230, 1–190, 1–154) and T7-tagged RORγt plasmid for 40 h, and co-immunoprecipitation using anti-Flag antibody from the cell extracts was performed and immunoblotted with anti-T7 antibody. Data are representative of three independent experiments. ( g ) 293T cells were co-transfected with an IL-17 promoter reporter construct containing the 6-kbp promoter, a RORγt plasmid and either a full-length IRF8 or the IRF8 truncation mutant (1–114) construct for 30 h. Luciferase assays were performed as described in b . Data indicate mean±s.d. of triplicate cultures and are representative of three independent experiments. * P <0.05 versus cells transfected with IRF8 mutant (Student's t -test). Full size image IRF8 controls T H 17-cell differentiation in vivo To further assess the effects of IRF8 on T H 17-cell differentiation in vivo , we performed adoptive transfer experiments using CD4 + CD62L + CD45RB hi CD25 – cells from WT and Irf8 –/– mice to induce colitis in RAG1 KO ( Rag1 –/– ) mice. Irf8 –/– mice did not develop spontaneous colitis during an observation period of 1.5 years ( Fig. 8a,b ). However, Rag1 –/– mice reconstituted with Irf8 –/– naive CD4 + T cells began losing weight earlier and lost more weight than mice in the control group. Parallel histological studies of colon sections from Rag1 –/– mice reconstituted with Irf8 –/– T cells revealed more severe inflammatory cell infiltrates and significantly higher pathological scores than those observed in sections from mice reconstituted with T cells from WT mice ( Fig. 8c–e ). In addition, mice reconstituted with Irf8 –/– cells had a significantly higher percentage of IL-17-producing cells than control mice ( Fig. 8f ). To determine whether T reg cells from Irf8 –/– mice could suppress effector T cells, we examined the population of T reg cells in Rag1 –/– mice after the transfer of naive WT or Irf8 –/– CD4 + T cells. Rag1 –/– recipients of naive CD4 + T cells from mice of either genotype generated a small percentage of CD4 + FOXP3 + and CD4 + IFN-γ + cells in the mesenteric lymph nodes ( Fig. 8f ). Furthermore, co-transfers of naive WT CD4 + T cells with CD4 + CD25 + cells purified from WT or Irf8 –/– mice resulted in similar effects on body weight ( Supplementary Fig. S9 ). These results indicate that the effects of IRF8 deficiency on T cell-mediated inflammation could not be explained by influences on the function of CD4 + T reg cells. Thus, IRF8 deficiency promotes intestinal inflammation in a T cell-mediated model of colitis, suggesting that IRF8 may have an inhibitory role in the control of T H 17-mediated immune responses. To further understand the role of IRF8 in T H 17-cell differentiation in vivo , we extended our observations to an infection model, as T H 17 cells have also been proposed to have a role in inflammation against both intracellular and extracellular bacteria [33] , [34] . Staphylococcus aureus is a Gram-positive bacterium that can induce IL-17 production from CD4 + T cells mainly through Staphylococcus aureus enterotoxin A (SEA), and humans deficient in T H 17 cells are highly susceptible to infection with this agent [35] , [36] . To better understand the regulatory effects of IRF8 on T H 17-cell differentiation in a broader sense, we used superantigenic S. aureus to induce IL-17 production in vivo . Spleen cells from Lck-Cre + Irf8 fl/fl and Lck-Cre + Irf8 wt/wt littermate controls immunized with SEA 4 days previously were re-stimulated in vitro with SEA for an additional 2 days and then examined for IL-17-producing CD4 + T cells by flow cytometry and for IL-17 secretion by ELISA ( Supplementary Fig. S10 ). IRF8-deficient mice generated significantly more IL-17-producing CD4 + T cells than WT mice, further confirming that IRF8 negatively regulates T H 17-cell differentiation in vivo . 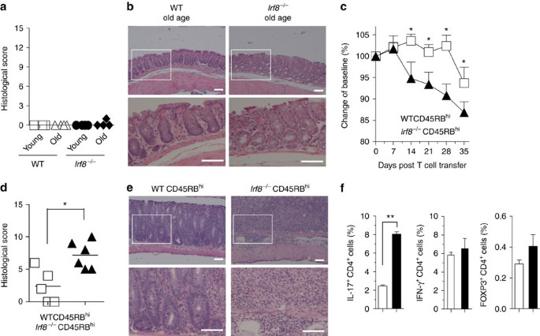Figure 8: Lack of IRF8 enhances the TH17 immune response in experimental colitis. WT andIrf8–/–mice were maintained under specific pathogen free (SPF). conditions for up to 18 months. Mice were killed and intestines were removed for histological analysis. Histology of colon tissues (a) and disease score (b) from age-matched young (15 weeks) and old (17–18 months) WT andIrf8–/–mice (three to four mice in each group). Scale bars, 200 μm. CD4+CD45RBhiT cells were purified from spleens and lymph nodes of wild-type orIrf8–/–mice and 5×105cells were injected (i.p.) into recipientRag–/–mice. Body weight change was monitored every week and mice were killed 7 weeks later. (c) Changes in body weight ofRag1–/–mice (n=5–6 mice per group) after intraperitoneal transfer of WT orIrf8–/–CD4+CD45RBhiT cells were recorded. Data are presented as the mean±s.d. of the percentage of initial body weight and are representative of two similar experiments. *P<0.05 versus recipients of WT cells (ANOVA test and Student'st-test). Disease scores (d) and sections of colons with colitis (e) fromRag1–/–mice (n=5–6 mice in each group) on day 35 after naive T cell transfer as described inc. *P<0.05 versus recipients of WT cells (Mann–Whitney test). Scale bars, 200 μm. (f) The percentage of IL-17, IFN-γ and FOXP3-producing cells from mesenteric lymph nodes ofRag1–/–mice inc(white column, transfer with WT cells; black column, transfer withIrf8–/–cells). **P<0.01 versus wild-type cell transferred mice (Student'st-test). Data are presented as the mean±s.d. from four mice in each group. Two independent experiments were performed with similar results. Figure 8: Lack of IRF8 enhances the T H 17 immune response in experimental colitis. WT and Irf8 –/– mice were maintained under specific pathogen free (SPF). conditions for up to 18 months. Mice were killed and intestines were removed for histological analysis. Histology of colon tissues ( a ) and disease score ( b ) from age-matched young (15 weeks) and old (17–18 months) WT and Irf8 –/– mice (three to four mice in each group). Scale bars, 200 μm. CD4 + CD45RB hi T cells were purified from spleens and lymph nodes of wild-type or Irf8 –/– mice and 5×10 5 cells were injected (i.p.) into recipient Rag –/– mice. Body weight change was monitored every week and mice were killed 7 weeks later. ( c ) Changes in body weight of Rag1 –/– mice ( n =5–6 mice per group) after intraperitoneal transfer of WT or Irf8 –/– CD4 + CD45RB hi T cells were recorded. Data are presented as the mean±s.d. of the percentage of initial body weight and are representative of two similar experiments. * P <0.05 versus recipients of WT cells (ANOVA test and Student's t -test). Disease scores ( d ) and sections of colons with colitis ( e ) from Rag1 –/– mice ( n =5–6 mice in each group) on day 35 after naive T cell transfer as described in c . * P <0.05 versus recipients of WT cells (Mann–Whitney test). Scale bars, 200 μm. ( f ) The percentage of IL-17, IFN-γ and FOXP3-producing cells from mesenteric lymph nodes of Rag1 –/– mice in c (white column, transfer with WT cells; black column, transfer with Irf8 –/– cells). ** P <0.01 versus wild-type cell transferred mice (Student's t -test). Data are presented as the mean±s.d. from four mice in each group. Two independent experiments were performed with similar results. Full size image T H 17 cells represent a recently defined member of a still growing family of T helper cells. The mechanisms involved in the silencing programme for this T helper subset remain unclear. Here we demonstrate that IRF8 serves as an intrinsic silencer for T H 17-cell differentiation. IRF8-deficiency in both conventional and T cell-specific conditional KO mice led to more robust T H 17-cell differentiation without effects on either T H 1 or T H 2 cell lineages. Furthermore, transfer of IRF8 –/– CD4 + CD45Rb hi cells into Rag1 –/– mice induced more severe colitis than transfer of WT CD4 + CD45Rb hi cells. In addition, mice reconstituted with IRF8 –/– cells had a significantly higher percentage of IL-17-producing cells than mice reconstituted with WT cells. In addition, we showed that IRF8 physically interacts with RORγt resulting in suppression of IL-17 transcription. These results suggest that IRF8 negatively regulates the development of T H 17 immune response resulting in the control of inflammation. Many studies have demonstrated that IRF8 has important functions in myeloid cells [24] . Macrophages from Irf8 –/– mice did not produce IL-12 in response to IFN-γ and LPS. IRF8 regulates IL-12 expression by binding to the IL-12 p40 promoter region, acting in synergy with IRF1 to activate IL-12 p40 gene expression [37] . In addition, IRF8 also induces the expression of other inflammatory proteins expressed by myeloid cells, including iNOS, IL-18 and IL-1 (refs 38 , 39 , 40 ). IRF8 protein levels are controlled in part by Cbl-mediated ubiquitylation and subsequent proteasomal degradation [41] . More recent studies have shown that transcriptional activation of IL-12p40 by IRF8 is enhanced following ubiquitylation by the E3 ubiquitin ligase, TRIM21 (ref. 42 ). Here, we showed that CD4 + T cells clearly expressed IRF8 protein on TCR engagement and that T H 17 polarization conditions induced stable IRF8 protein expression. In addition, mitogen-activated protein kinase inhibitors completely blocked IRF8 protein expression induced by TCR activation and STAT3 mutant mice showed impaired IRF8 mRNA expression, indicating that the TCR signalling cascade is involved in induction of IRF8 expression. The percentages of CD4 + T cells in tissues of Irf8 –/– and WT mice were comparable. Following stimulation under T H 17 polarizing conditions, however, the percentages of IL-17-producing CD4 + T cells were greatly increased and the expression of T H 17 signature genes was significantly enhanced for cells from Irf8 –/– as compared with WT mice. These results suggest that IRF8 is an important transcription factor in controlling CD4 + T cell plasticity by targeting T H 17-cell differentiation. The balance between pathogenic T H 17 cells and suppressive T reg cells in the immune system depends on the presence of inflammatory cytokines such as IL-6 and IL-21 (ref. 43 ). The anti-inflammatory cytokine, TGF-β, combined with IL-6 or IL-21 can drive the conversion of a T H cell phenotype from TGF-β-induced FOXP3-expressing T reg cells to RORγt-expressing T H 17 cells. TGF-β inhibits the expression of STAT4 and GATA3, thereby preventing the differentiation of T H 1 and T H 2 cells, respectively, and concurrently facilitating T H 17-cell development. CD4 + T cells from WT and Irf8 –/– mice yielded similar populations of FOXP3 + cells following stimulation under T H 17- or T reg -inducing conditions. In addition, there were no significant differences between WT and Irf8 –/– T H 17 cells in the production of the autocrine cytokines, IL-21 and IL-10. These results rule out the possibility that enhanced generation of T H 17 cells by CD4 + T cells from Irf8 –/– mice stimulated with TGF-β plus IL-6 was due to alterations in TGF-β-derived T reg suppression or to an autocrine loop involving IL-21 or IL-10. IRF8 acts as a transcriptional repressor or a transcriptional activator depending on the target DNA sequence and interactions with different partner proteins, including PU.1, E47 and other IRFs [25] . We demonstrated that IRF8 interacts directly with RORγt, resulting in suppression of IL-17 transcription. The association of IRF8 with RORγt was not competed by FOXP3, another RORγt-binding protein [44] , indicating that IRF8 antagonizes the effect of RORγt without the involvement of FOXP3. In addition, co-immunoprecipitation studies showed that IRF4, another IRF family member required for T H 17-cell differentiation [32] , also interacts with RORγt. It is likely that RORγt cooperates with other transcription factors, such as FOXP3 or RUNX1, or unknown factors in the regulation of T H 17 differentiation [26] , [29] , [30] . It remains to be determined how these factors might collaborate with RORγt, the master transcription factor for T H 17 cells to regulate differentiation of this T H subset. T H 17 cells are critical pathogenic effector T cells in inflammatory disorders such as inflammatory bowel disease [45] , [46] , [47] . In the present study, we demonstrated that IRF8 targets RORγt, resulting in the silencing of T H 17-cell differentiation. In addition, transfer of IRF8 –/– CD4 + CD45Rb hi cells into Rag1 –/– mice induced more severe colitis than transfer of WT cells. These results suggest that IRF8 functions as an important transcription factor in the control of inflammation by modulating RORγt activity. A recent genome-wide association study identifying IRF8 as a susceptibility locus in patients with multiple sclerosis [48] is supportive of this model for IRF8 function in inflammatory diseases. As a result, our data may provide a molecular basis for identifying specific single-nucleotide polymorphisms associated with susceptibility to clinical immune pathologies. Taken together, our results demonstrate that IRF8 is stably expressed during T H 17-cell differentiation and has a critical role in directing the silencing programme for T H 17-cell development. On the basis of these studies, we propose a novel molecular mechanism for the inhibitory effects of IRF8 on T H 17 differentiation and cytokine expression that involves the modulation of RORγt activity ( Supplementary Fig. S11 ). Our observations support a pathogenic role for T H 17 cells in exacerbating inflammation and indicate that IRF8 may be a therapeutic target for controlling T H 17-mediated autoimmune and inflammatory diseases. Mice C57BL/6 (B6) and B6- Irf8 –/– mice were maintained in the barrier facility at the Mount Sinai School of Medicine. GFP-FOXP3 mice were crossbred with Irf8 –/– mice to obtain Irf8 –/– GFP-FOXP3 mice. IRF8 conditional knockout mice ( Irf8 fl/fl ) were generated at Ozgene under a contract with NIAID by flanking exon 2 and an inserted PGK-neo cassette with loxP sites. Following homologous recombination of the targeting vector in C57BL/6 ES cells and establishment of germ line transmission, the PKG-neo cassette, which was flanked by flippase recognition target (FRT) sites, was excised by crossing with a FLP transgenic mouse. Selective breeding was used to eliminate the FLP gene. Conditional deletion of IRF8 in T cells was performed by crossing with Lck-Cre mice to generate Lck-Cre + Irf8 fl/fl mice. The animal study protocols were approved by the Institutional Animal Care and Use Committees of Mount Sinai, NICHD and NIAID (protocol LIP-4). Antibodies The following antibodies were purchased from BD Biosciences, as conjugated to FITC, PE, PE-Cy5, perCP-Cy5.5 or APC: CD4 (L3T4), CD8 (53-6.7), CD3e (145-2C11), CD25 (PC61.5), CD44 (IM7), CD62L (MEL-14), CD45RB (C363-16A), IL-17 (TC11-18H10), IFN-γ (XMG1.2), TCRβ chain (H57-597) and isotype controls. Antibodies for IL-2 (JES6-1A12), IL-4 (11B11), IL-10 (JES5-16E3) and Foxp3 (FJK-16S) were purchased from eBiosciences. CD4 + T cell preparation and differentiation in vitro Naive CD4 + T cells (CD62L + CD44 lo ) were prepared by fluorescence-activated cell sorting from spleens and lymph nodes of Irf8 –/– and WT littermates. The sorted cells were primed for 96 h with anti-CD3 (1 μg ml −1 ; 145-2C11; BD Biosciences) and soluble anti-CD28 (2 μg ml −1 ; 37.51; BD Biosciences). The cells were rested for 48 h, and were then re-stimulated for 5 h with PMA plus ionomycin in the presence of brefeldin A and intracellular cytokines were measured by flow cytometry. Cells stimulated under neutral conditions were defined as T H 0 cells. Cells were stimulated to differentiate into T H 1 cells by supplementation with IL-12 plus anti-IL-4 (10 μg ml −1 ; 11B11; BD Bioscences) or into T H 2 cells by supplementation with IL-4 and anti-IFN-γ (10 μg ml −1 ; XMG1.2, BD Biosciences). For T H 17-cell differentiation, cells were stimulated with transforming growth factor-β1 (5 ng ml −1 ), IL-6 (20 ng ml −1 ) and IL-23 (10 ng ml −1 ; all from R&D Systems) in the presence of anti-IL-4 antibody (10 μg ml −1 ; 11B11, BD Bioscences) and anti-IFN-γ antibody (10 μg ml −1 ; XMG1.2, BD Biosciences). Intracellular staining and flow cytometry Cells were stimulated with PMA and ionomycin for 5 h in the presence of brefeldin A before intracellular staining. Cells were fixed with IC Fixation Buffer (BD Biosciences), incubated with permeabilization buffer, and stained with PE-anti-mouse IL-17, APC-anti-IFN-γ and PE-Cy 5.5 anti-mouse CD4 antibodies. Flow cytometry was performed on a FACSCalibur (BD Biosciences) and LSR Fortessa (BD Biosciences). RNA isolation and quantitative real-time RT–PCR Total RNA was extracted using an RNeasy plus kit (QIAGEN) and cDNA was generated with an oligo (dT) primer and the Superscript II system (Invitrogen) followed by analysis using iCycler PCR with SYBR Green PCR master Mix (Applied Biosystems). Results were normalized based on the expression of ubiquitin. The following primer sets were used: IL-17A, IL-17F, IL-21, IL-23R, RORγt, IFN-γ, IRF8, IRF1 IRF4 T-bet FOXP3, CCR6, IL-10, IL-4, IL-2 and ubiquitin ( Supplementary Table S1 ). Transfection and luciferase reporter assay 293T cells were transiently transfected with an IL-17 promoter luciferase reporter plasmid together with RORγt in the presence of IRF8 plasmid at different concentrations. For each transfection, 2.0 μg of plasmid was mixed with 100 μl of Opti-MEM I medium (without serum and antibiotics) and 4.0 μl of Lipofectamine 2000 reagent. The mixture was incubated at room temperature for 20 min and added to 12-well plates containing cells and complete medium. The cells were incubated for 30 h and collected using reporter lysis buffer (Promega) for determination of luciferase activity. Cells were co-transfected with a β-galactosidase reporter plasmid to normalize experiments for transfection efficiency. Generation of the mutant IL-17 promoters A predicted IRF-binding site adjacent to the downstream RORγt-binding site in the CNS2 region of the mouse IL-17A promoter was mutated using QuickChange XL Site-Directed Mutagenesis Kit (Stratagene) according to manufacture's instruction. Two mutations were introduced on the IL-17 promoter regions −5204 to −5202 (TGG to CCC) and −5201 to −5199 (AAA to CCC) from the transcriptional initiation site (+1) using the following primer sets: 5′-GGTTGGAAAAAAAAA CCC AAAGTTTTCTGACCCA-3′ and 5′-TGGGTCAGAAAACTTGGGTTTTTTTTTCCAACC-3′ for TGG to CCC; 5′-TGGAAAAAAAAATGG CCC GTTTTCT-GACCCACT-3′ and 5′-AGTGGGTCAGAAAACGGGCCATTTTTTTTTCCA-3′ for AAA to CCC. Mutations were verified by sequencing. Retroviral transduction of IRF8 in CD4 + T cells To prepare pseudotyped virus human 293 EbnaT cells were seeded at a density of 4×10 6 cells in a 10-cm dish. The next day, cells were transfected using calcium phosphate with a mixture of 2.5 μg of plasmid pMD.G encoding vesicular stomatitis virus G protein, 7.5 μg of plasmid encoding gag-pol, and 10 μg of a retroviral expression constructs encoding GFP or IRF8. At 48 h after transfection, the viral supernatant was collected, centrifuged at 800 g , and used to infect cells. CD4 + T-cell transduction was performed as previously described [11] , sorted naive CD4 + T cells were plated as above and cultured for 24 h in the presence of anti-CD3 (1 μg ml −1 ; 145-2C11, BD Biosciences) and soluble anti-CD28 (2 μg ml −1 ; 37.51; BD Biosciences). Activated cells were then transduced with fresh retrovirus supernatant by centrifugation for 1.5 h at 2000 g in the presence of polybrene (6 μg ml −1 ; Sigma). After 24 h, the cells were re-transduced using the same procedure and cultured for an additional 24 h and were then stimulated with TGF-β and IL-6. The cells were collected on day 5 or 6 for intracellular cytokine staining. T-cell proliferation assay Naive CD4 + T cells were purified from spleens and lymph nodes of Lck-Cre + Irf8 fl/fl and Lck-Cre + Irf8 wt/wt littermate controls. Cells (1×10 5 per well) were cultured in the absence or presence of anti-CD3 (1 μg ml −1 ) and anti-CD28 (2 μg ml −1 ) antibodies for 3 days in 96-well microplates. [ 3 H]-Thymidine was added during the last 8 h of a 72-h culture. The cells were then collected and counted with a beta-counter. Co-immunoprecipitation and immunoblotting analysis Cells were washed with cold phosphate-buffered saline and lysed for 15 min on ice in 0.5 ml of lysis buffer (50 mM Tris-HCl, pH 8.0, 280 mM NaCl, 0.5% Nonidet P-40, 0.2 mM EDTA, 2 mM EGTA, 10% glycerol and 1 mM dithiothreitol) containing protease inhibitors. Cell lysates were clarified by centrifugation (4 °C, 15 min, 20,000 r.p.m. ), aliquots (500 μg) were incubated with 2 μg of normal rabbit IgG for 4 h and 20 μl of protein G-Sepharose was added to the mixture for 2 h. After centrifugation, the supernatant was collected and incubated with 2 μg of anti-Flag antibody overnight at 4 °C with gentle rocking, after which immune complexes were collected as described above with 20 μl of protein G-Sepharose. After washing five times with lysis buffer, immunoblotting was performed. Anti-Flag (Sigma), anti-IRF8 (Santa Cruz), anti-β-actin (Sigma) and anti-T7 (MBL) antibodies were used according to the manufactures' instructions. Secondary antibodies were from Santa Cruz. T-cell-transfer colitis studies and histopathology T-cell-transfer colitis was performed as previously described [49] , [50] . Briefly, purified CD4 + CD45RB hi T cells from WT and Irf8 –/– mice were injected intraperitoneally into Rag1 –/– recipients (5×10 5 cells per mouse in 200 μl sterile PBS per injection). Mice were weighed every week throughout the course of experiments. After 5 weeks, mice were killed and colon tissues were excised. Tissues were fixed in 10% buffered formalin and paraffin embedded. The sections (5 μm) of tissue samples stained with hematoxylin and eosin. All the slides were read and scored by an experienced pathologist (L.Q.) without previous knowledge of the type of treatment. The degree of inflammation in the epithelium, submucosa and muscularis propria was scored separately as described by Totsuka et al . [49] In vivo stimulation of T H 17 cells by Staphylococcus aureus Lck-Cre + Irf8 fl/fl mice and Lck-Cre + Irf8 wt/wtl littermate controls were immunized (i.p.) with SEA (10 μg per mouse) for 4 days. Mice were killed and spleen cells were prepared. The cells were re-stimulated in vitro with SEA (10 ng ml −1 ) for additional 2 days and cells were collected for the analysis of IL-17-producing CD4 + T cells by flow cytometry gating on CD4 + T cells. The supernatants were collected for the measurement of IL-17 production by ELISA. Chromatin immunoprecipitation assay The ChIP procedure was performed using an assay kit following the manufacturer's instruction (Upstate Biotechnology). Briefly, 293T cells were co-transfected with an IL-17 promoter containing CNS2 domain and an IRF8 plasmid for 36 h and 1×10 7 transfected cells were then crosslinked by 1% formaldehyde for 10 min at 37 °C. Nuclei were prepared and subjected to sonication to obtain DNA fragments. Chromatin fractions were precleared with protein A-agarose beads followed by immunoprecipitation overnight at 4 °C with 3 μg of anti-IRF8 or control antibody. Crosslinking was reversed at 65 °C for 4 h, followed by proteinase K digestion. DNA was purified and subjected to qPCR. The input DNA was diluted 200 times before PCR amplification. The input and immunoprecipitated DNA were amplified by qPCR using primers (5′-CAGCCCTGGTCCTTAAACTG-3′ and 5′-TCACTTTCGTTGTGCCTTTG-3′) encompassing the CNS2 region of the mouse IL-17 promoter. Cytokine ELISA Supernatants from cell cultures were collected after activation under various conditions and secreted cytokines in the supernatants were measured by ELISA kits with purified coating and biotinylated detection antibodies: anti-IL-17, anti-22 and anti-IL-21 (R&D systems), anti-IFN-γ, anti-IL-4 and anti-IL-10 (BD Bioscience). Statistical analysis Statistical analysis was performed using Student's t -test for most of the experiments. For colitis experiments, Man–Whitney test and analysis of variance test were used for comparison of disease score and weight loss. P values <0.05 were considered statistically significant. How to cite this article: Ouyang, X. et al . Transcription factor IRF8 directs a silencing programme for T H 17-cell differentiation. Nat. Commun. 2:314 doi: 10.1038/ncomms1311 (2011).